Semiconductor/relaxor 0–3 type composites without thermal depolarization in Bi0.5Na0.5TiO3-based lead-free piezoceramics Commercial lead-based piezoelectric materials raised worldwide environmental concerns in the past decade. Bi 0.5 Na 0.5 TiO 3 -based solid solution is among the most promising lead-free piezoelectric candidates; however, depolarization of these solid solutions is a longstanding obstacle for their practical applications. Here we use a strategy to defer the thermal depolarization, even render depolarization-free Bi 0.5 Na 0.5 TiO 3 -based 0–3-type composites. This is achieved by introducing semiconducting ZnO particles into the relaxor ferroelectric 0.94Bi 0.5 Na 0.5 TiO 3 –0.06BaTiO 3 matrix. The depolarization temperature increases with increasing ZnO concentration until depolarization disappears at 30 mol% ZnO. The semiconducting nature of ZnO provides charges to partially compensate the ferroelectric depolarization field. These results not only pave the way for applications of Bi 0.5 Na 0.5 TiO 3 -based piezoceramics, but also have great impact on the understanding of the mechanism of depolarization so as to provide a new design to optimize the performance of lead-free piezoelectrics. Piezoelectric materials are indispensable in daily life because they have wide applications in electromechanical devices such as sensors, actuators and so on. Up to now, the most dominantly commercialized piezoelectric materials contain lead exemplified by lead–zirconate–titanate-based materials, but lead is toxic to human health and the environment. Therefore, with the enforcement of regulations on the restriction of the use of hazardous substances in electronic devices [1] , [2] , intensive efforts have been continuously devoted to the search for lead-free replacement and to the understanding of the enhancement mechanisms for piezoelectric behaviour [3] , [4] , [5] , [6] , [7] , [8] . There has been a steady progress on the development of lead-free piezoelectrics. Many lead-free piezoelectric materials have been reported, consisting mostly of solid solutions with morphotropic phase boundary compositions based on BaTiO 3 (BT), K 0.5 Na 0.5 NbO 3 (KNN) and Bi 0.5 Na 0.5 TiO 3 (BNT). However, it is still not possible to completely replace lead–zirconate–titanate materials due to a common drawback concerning the phase transition of these lead-free materials. The BT-based solid solutions are limited due to the low Curie temperature ( T c ), which is around 120 °C. KNN-based solid solutions also have a similar problem, its giant piezoelectric property happens at the transition between orthorhombic and tetragonal structure ( T O–T ). This transition is composition sensitive and the transition temperature can be tuned down to near room temperature (RT). These drawbacks, limiting the working temperature and affecting the property’s temperature stability, are difficult to overcome. Thus they hinder the application of BT- and KNN-based lead-free materials [6] , [9] , [10] , [11] . As one of the most feasible lead-free candidates, BNT-based solid solutions have good piezoelectric property, excellent reproducibility and high maximum dielectric constant temperature ( T m ~300 °C) [4] , [5] , [6] . However, its most noticeable drawback is the depolarization at around 100 °C ( T d ), which is much lower than the T m (300 °C) [4] , [6] , [12] , [13] , [14] . This thermal depolarization leads to the disappearance of macroscopic piezoelectric behaviour so that the T d determines the upper-limit working temperature. If the thermal depolarization could be suppressed or eliminated, the path to application of these lead-free piezoceramics would be open. A large amount of attempts using conventional methods based on solid solution or chemical doping have been explored, but failed to suppress or eliminate the depolarization of BNT-based solid solutions. Such methods generally lead to decreased T d towards RT to enhance RT piezoelectric properties [12] , [15] , [16] , [17] , while the increase on T d is at the expense of reduced piezoelectric properties. Up to now, it is still a challenge to increase T d and enhance piezoelectric properties simultaneously. Therefore, an alternative method must be developed to resolve this problem. Here we report the composites of 0.94Bi 0.5 Na 0.5 TiO 3 –0.06BaTiO 3 : x ZnO (BNT–6BT: x ZnO), which show excellent piezoelectric properties without depolarization and enhanced temperature stability. The parameter x (0~0.4) represents the mole ratio of ZnO over BNT–6BT. Perovskite BNT–6BT ceramic is well known to have a rhombohedral-tetragonal morphotropic phase boundary and demonstrates good electromechanical properties [18] . Wurtzite ZnO is a polar semiconductor with piezoelectricity [19] , [20] , [21] . BNT–6BT and ZnO have only limited solid solution and hence afford the formation of composites. To highlight the specific nature of ZnO, composites formed by the same matrix BNT–6BT, but different oxide ZrO 2 (a typical dielectric insulator [22] ) are prepared and investigated. Phase and microstructure analysis The X-ray diffraction (XRD) patterns ( Supplementary Fig. 1 ) reveal that the samples with x =0.2, 0.3 and 0.4 have two sets of diffractions peaks from BNT–6BT and ZnO, which indicate that these samples are composites instead of solid solutions. XRD measurements on both unpoled and poled samples ( Supplementary Fig. 2a,b ) reveal that composites with higher ZnO content retain the poled state, as confirmed by the poling-induced tetragonal structure, indicated by splitting of the diffraction peak around 2 θ ~46.5° (ref. 23 ). Further temperature-dependent XRD patterns on poled samples with x =0.3 ( Supplementary Fig. 2c ) and 0.4 prove that such a poled state is stable up to ~240 °C, which is close to the T m . It indicates the absence of thermal depolarization, as will be discussed in more detail below. Furthermore, different grain ensembles in the compositions with x =0.3 and 0.4 also indicate the composite structure ( Supplementary Fig. 3 ). To reveal the composition visually, a typical two-dimensional element mapping of x =0.3 is demonstrated in Fig. 1a . Three features are noticeable. First, there are two sets of grains corresponding to BNT–6BT and ZnO, respectively. We suggest that there is limited cation diffusion between BNT–6BT and ZnO, since the solution limit is very low [24] , [25] . Some Zn ions have entered into the lattice as the sintering is enhanced and the grain size becomes larger with increasing ZnO content ( Supplementary Fig. 3 ). Second, the initially nano-sized ZnO (25 nm) has grown into larger ZnO particles with the average size of ~500 nm. Most of the irregular ZnO particles are located at boundaries between BNT–6BT grains. Third, 0–3-type composites have been formed, in which the BNT–6BT grains form a three-dimensional network, while the ZnO particles are isolated. Note that each BNT–6BT grain has several neighbouring and independent ZnO particles. For further confirmation, the detailed element distribution and the energy-dispersive spectrum recorded from the same area are provided in Fig. 1b . Obvious chemical inhomogeneity is observed: the Ba, Ti and Na cations occupy the same areas and these areas connect with each other, whereas Zn cations occupy the remaining and isolated areas. 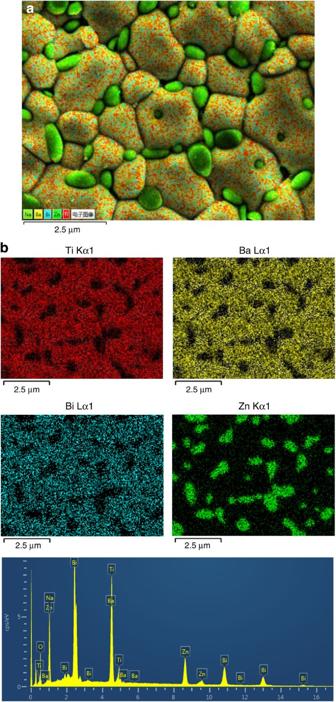Figure 1: SEM micrographs of BNT–6BT:0.3ZnO. (a) The microstructure image reveals the ZnO particles and BNT–6BT grains forming a 0–3-type composite structure. Scale bar, 2.5 μm. (b) The corresponding element distribution and energy-dispersive spectrum pattern recorded from the local area further confirm the composite structure. Figure 1: SEM micrographs of BNT–6BT:0.3ZnO. ( a ) The microstructure image reveals the ZnO particles and BNT–6BT grains forming a 0–3-type composite structure. Scale bar, 2.5 μm. ( b ) The corresponding element distribution and energy-dispersive spectrum pattern recorded from the local area further confirm the composite structure. Full size image The theoretical volume fraction of ZnO in the composite of BNT–6BT: x ZnO can be calculated by considering the theoretical densities of BNT–6BT and ZnO. The theoretical volume fractions of ZnO are calculated to be 5.3%, 11.9%, 20.5% and 31.9% for the compositions with x =0.1, 0.2, 0.3 and 0.4, respectively. The experimental volume fraction of ZnO can be basically quantified according to the area ratio of different components provided in the scanning electron micrograph (SEM) ( Fig. 1a ). For compositions with small amount of ZnO ( x =0.1 and 0.2), the volume fraction cannot be experimentally determined from SEM because no clear ZnO particles can be observed. For x =0.3 and 0.4, the volume fractions of ZnO are calculated to be ~13% and 24%, respectively. The relatively lower experimental volume fraction values of ZnO compared with theoretical values could be attributed to the fact that not all initial 25-nm-sized ZnO particles have grown into large particles. Such an 0–3-type composite structure has also been confirmed by micro-Raman measurements, which were carried out on the four grains labelled as grain 1, grain 2, grain 3 and grain 4 ( Supplementary Fig. 4a ). The Raman spectrum of each grain is plotted in Supplementary Fig. 4b . The mode at ~439 cm −1 coming from ZnO (ref. 26 ) can only be observed in grain 1, grain 2 and grain 3. The other modes at ~286, ~534 and ~608 cm −1 attributed to BNT–6BT [13] , [27] are not dependent on the ZnO concentration, indicating that the introduction of ZnO has not changed the crystal structure of the BNT–6BT matrix. Hence, ZnO and BNT–6BT are independent of each other in forming the 0–3-type composite structure, which is further confirmed by the two-dimensional Raman spectrum mapping with the fixed mode of 286 cm −1 , as depicted in Supplementary Fig. 4c . Temperature-dependent dielectric constant and loss The temperature-dependent dielectric constant ( ε r ) and loss (tan δ ) of all compositions measured at 1 kHz are contrasted in Fig. 2a,b , respectively. The curves of the composition with x =0 are consistent with previous reports [13] , [26] . The first anomaly of dielectric constant or the sharp decrease of dielectric loss around 100 °C is attributed to the depolarization behaviour, which is an indication for T d [5] , [13] , [26] , [27] , [28] . As can be seen, with increasing ZnO concentration from 0 to 0.2, the T d increases from ~98 °C for x =0 to ~130 °C for x =0.1, and to ~150 °C for x =0.2, indicating the progressively suppressed thermal depolarization. More interestingly, with further increasing ZnO concentration to 0.3 and 0.4, the first anomaly of dielectric constant and the sharp decrease of dielectric loss disappear, indicating the completely eliminated thermal depolarization. At the same time, the peak of dielectric loss for both compositions appears around 245 °C, close to T m (~280 °C). The peak temperature determined from dielectric loss is slightly lower than that from the dielectric constant, which is attributed to the relaxor nature in the BNT system [29] . Note that the absence of the depolarization in the present composites has not been reported in any BNT-based or other lead-free materials. One may bear in mind that the possibility of an increase in T d by forming solid solution between Zn cations and the BNT–BT lattice could be excluded due to the fact that T d is reduced by the chemical Zn substitution [25] . For a succinct mechanistic understanding, the compositional dependence of permittivity on composition may be of interest. However, we are not only contemplating a complex rule of mixtures, but also expect that the domain structure responds to the altered local electric fields, which complicates a further discussion. 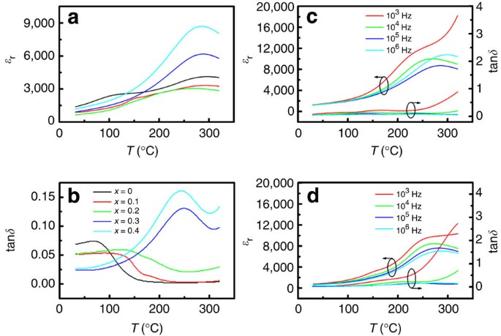Figure 2: Temperature-dependent dielectric property. (a) Dielectric constant and (b) dielectric loss of all samples measured at 1 kHz. The disappearance of the first anomaly of dielectric constant and the sharp decrease of dielectric loss around 100 °C in the compositions withx=0.3 and 0.4 are clearly observed, indicating the absence of depolarization. Both (c) unpoled and (d) poled BNT–6BT:0.3ZnO show no thermal depolarization at all measuring frequencies. Figure 2: Temperature-dependent dielectric property. ( a ) Dielectric constant and ( b ) dielectric loss of all samples measured at 1 kHz. The disappearance of the first anomaly of dielectric constant and the sharp decrease of dielectric loss around 100 °C in the compositions with x =0.3 and 0.4 are clearly observed, indicating the absence of depolarization. Both ( c ) unpoled and ( d ) poled BNT – 6BT:0.3ZnO show no thermal depolarization at all measuring frequencies. Full size image For more detailed information on dielectric property, the temperature-dependent ε r and tan δ of all unpoled compositions are measured at different frequencies. Typical results of the x =0.3 composition are plotted in Fig. 2c . The most noticeable feature is that the well-known anomalies of ε r and tan δ corresponding to T d disappear at all measuring frequencies. For example, there is only one anomaly of ε r around 280 °C, indicating the absence of depolarization in this composition. The frequency-dependent ε r points to the relaxor nature of the composition, due to the coexistence of R3c and P4bm phases of BNT–6BT [30] , [31] . The dielectric property measured on the poled composition of x =0.3 is plotted in Fig. 2d for comparison. For BNT-based solid solutions, if the temperature-dependent ε r and tan δ are measured on poled samples, the ε r and tan δ peaks corresponding to T d should be observed [31] ; however, such peaks are absent in Fig. 2d , which further confirms the absence of depolarization in the composite. Composition-dependent ferro- and piezoelectric properties at RT To optimize the property, the compositions of BNT–6BT: x ZnO with the x -value of 0–0.6 were prepared. It has been found that the resistivity decreased significantly when the ZnO content was greater than 0.4, especially for x =0.6. RT polarization–electric-field ( P–E ) loops, bipolar and unipolar strain–electric-field ( S–E ) curves of the BNT–6BT: x ZnO ( x =0~0.4) are plotted in Fig. 3a–e . The corresponding composition-dependent saturated polarization ( P s ) and remnant polarization ( P r ), and piezoelectric coefficient ( d 33 ) of x =0~0.5 are depicted in Fig. 3f . Three important features are emphasized as follows. (1) All compositions have well-shaped P–E loops and butterfly-shaped bipolar S–E curves, indicating a typical ferroelectric nature at RT. The P s , P r and d 33 values increase with increasing x . Note that the P s , P r and d 33 values of the composites are larger than other reported values of pure BNT–6BT ceramics [27] , [32] , but lower than corresponding values in single crystals [33] . This is related to the charge-compensating effect of ZnO as discussed below. A further confirmation is provided by the fact that the P–E loops provide a more rectangular shape with limited back-switching, when the electric field is removed, particularly with x =0.3 and 0.4. (2) For each composition, the applied electric field is close to the electric breakdown field. For example, for the BNT–6BT:0.3ZnO, the measuring field is 12 kV mm −1 . The ceramic will feature dielectric breakdown if the field is increased further. So, the breakdown field is 6, 10, 10, 12, 17 and 12 kV mm −1 for x =0~0.5, respectively. It is interesting to observe that the breakdown field of BNT–6BT:0.4ZnO composite is ~3 times higher than that of single-phase BNT–6BT. So, the breakdown strength has been greatly improved by the introduction of ZnO. The increase of breakdown strength as ZnO content increases is mainly due to ZnO-improved relative density or the reduction of porosity ( Supplementary Fig. 3 ). Furthermore, we suggest that the ZnO partially compensates the depolarization field and therefore smoothens the intrinsic electric field distribution. (3) The electric properties degrade when x reaches 0.5, where wide-scale percolation of the ZnO is reached. 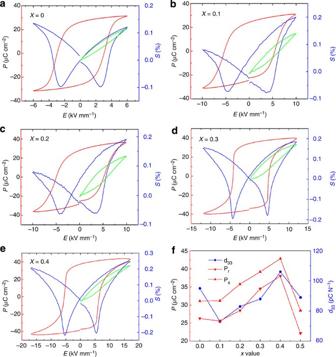Figure 3: Composition-dependent room-temperature ferroelectric and piezoelectric properties. (a–e) Bipolar P-E loops (red), bipolar S-E curves (blue) and unipolar S-E curves (green). The well-shapedP–Eloops and butterfly-like bipolarS–Ecurves confirm the ferroelectric nature of these compositions. Also, the breakdown field increases from 6 kV mm−1forx=0, to 10 kV mm−1forx=0.1 and 0.2, 12 kV mm−1forx=0.3 and 17 kV mm−1forx=0.4. (f) The composition dependences ofPs,Prandd33clearly indicate that ZnO can enhance both ferroelectric and piezoelectric properties. Whenxreaches 0.5, the electric properties tend to decrease as the content of ZnO has passed the percolation threshold. Figure 3: Composition-dependent room-temperature ferroelectric and piezoelectric properties. ( a – e ) Bipolar P-E loops (red), bipolar S-E curves (blue) and unipolar S-E curves (green). The well-shaped P–E loops and butterfly-like bipolar S–E curves confirm the ferroelectric nature of these compositions. Also, the breakdown field increases from 6 kV mm −1 for x =0, to 10 kV mm −1 for x =0.1 and 0.2, 12 kV mm −1 for x =0.3 and 17 kV mm −1 for x =0.4. ( f ) The composition dependences of P s , P r and d 33 clearly indicate that ZnO can enhance both ferroelectric and piezoelectric properties. When x reaches 0.5, the electric properties tend to decrease as the content of ZnO has passed the percolation threshold. Full size image It should be emphasized that the P–E loops provided in Fig. 3 are measured with different applied electrical fields. This is required as the coercive field is enhanced with increasing ZnO content. If measured with the same electric field, for example, 6 kV mm −1 , the P s and P r decrease from x =0 to 0.2, then increase for x =0.3 and 0.4 ( Supplementary Fig. 5 ). We hypothesize that there are two competing effects of ZnO on the measured values of ferroelectric parameters: one is that ZnO and BNT–6BT obey polarization (connection in series) and strain (connection in parallel) coupling [34] ; this leads to a reduced local electric field in the BNT–6BT and to overall decreased P s and P r values. The other is that ZnO bolsters ferroelectricity by retaining the tetragonal phase after poling ( Supplementary Fig. 2 ), which could increase P s and P r values. Accordingly, the reduction of P s and P r in x =0.1 and 0.2 samples is attributed to the fact that the positive effects of ZnO to enhance P s and P r is less dominant, whereas it becomes predominant in the compositions with higher Zn content ( x =0.3 and 0.4). Temperature-dependent ferro- and piezoelectric properties Figure. 4a–e plots the temperature-dependent P–E loops and current–electric-field ( J–E ) curves of the BNT–6BT:0.3ZnO composite, while Fig. 4f demonstrates the temperature-dependent P s , P r and E c . The two peaks in the J–E curves are due to the polarization-switching current. From 25 to 125 °C, the well-shaped ferroelectric P–E loops and J–E curves confirm the ferroelectric nature. Furthermore, P s and P r are almost temperature independent, except for a strong increase around 125 °C arising from thermally induced leakage. The E c decreases monotonously with increasing temperature. For comparison, temperature-dependent P–E loops and J–E curves of BNT–6BT without the addition of ZnO are provided in Fig. 5a–e . The slightly pinched P–E loops and four-peak J–E curves indicate that this solid solution tends to depolarize near 50 °C, consistent with previous reports [27] , [30] . In such case, the P s is almost temperature independent, whereas the P r decreases sharply above 50 °C ( Fig. 5f ). By comparing the results plotted in Figs 4 and 5 , it is reasonable to conclude that the BNT–6BT:0.3ZnO composite is free from depolarization and exhibits improved ferroelectric property and thermal stability of the composite. A key to further discussions may be that the switching currents of the composite materials have a narrower distribution as compared with the materials without the ZnO. Note that the composite of BNT–6BT:0.4ZnO has similar temperature-independent P–E and J–E curves as that of BNT–6BT:0.3ZnO, but has increased leakage ( Supplementary Fig. 6 ). 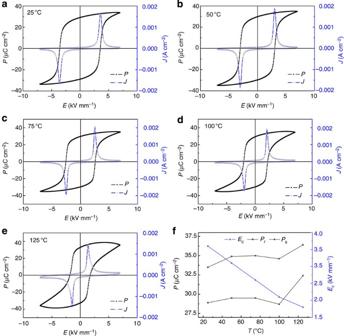Figure 4: Temperature-dependentP–Eloops andJ–Ecurves of BNT–6BT:0.3ZnO composite. (a–e) These results confirm the ferroelectric nature of this composite; no depolarization behaviour can be detected in the temperature range from 25 to 125 °C. (f) The corresponding temperature dependences ofPs,PrandEc. Obviously, the temperature stability of ferroelectric properties has been improved in the composite. Figure 4: Temperature-dependent P–E loops and J–E curves of BNT–6BT:0.3ZnO composite. ( a – e ) These results confirm the ferroelectric nature of this composite; no depolarization behaviour can be detected in the temperature range from 25 to 125 °C. ( f ) The corresponding temperature dependences of P s , P r and E c . Obviously, the temperature stability of ferroelectric properties has been improved in the composite. 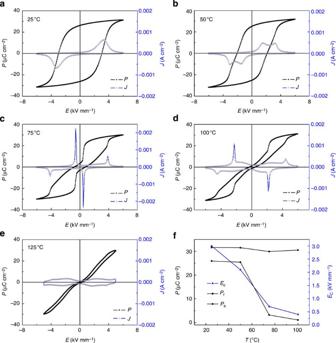Figure 5: Temperature-dependentP–Eloops andJ–Ecurves of BNT–6BT solid solution. (a–e) The appearance of ‘pinched’P–Eloops and ‘four-peak’J–Ecurves near 50 °C confirm the onset of depolarization. (f) The temperature-dependentPs,PrandEcreveal that the ferroelectricity of this solid solution is temperature sensitive, which is due to the existence of depolarization. Full size image Figure 5: Temperature-dependent P–E loops and J–E curves of BNT–6BT solid solution. ( a – e ) The appearance of ‘pinched’ P–E loops and ‘four-peak’ J–E curves near 50 °C confirm the onset of depolarization. ( f ) The temperature-dependent P s , P r and E c reveal that the ferroelectricity of this solid solution is temperature sensitive, which is due to the existence of depolarization. Full size image The bipolar and unipolar S – E curves of BNT–6BT:0.3ZnO were also measured at different temperatures ( Fig. 6a–e ). If we define the total strain as the difference between positive and negative maximum strain, and define the negative strain as the difference between the zero-field strain and the lowest strain, then the temperature-dependent total strain, negative strain, maximum unipolar strain, and maximum unipolar strain/maximum electric field ( S max / E max ), which is the large signal d 33 ( d 33 *) (ref. 6 ), are plotted in Fig. 6f . The comparative results of BNT–6BT are provided in Fig. 7 . It has been reported that at around T d , the negative strain tends to be zero in the bipolar S – E curves, while the unipolar S – E curves tend to have large recoverable strain with large hysteresis because of the loss of ferroelectric order [14] , [15] , [27] , [34] , which is consistent with the results near 75 °C (see Fig. 7 ). However, it is not the case in the BNT–6BT:0.3ZnO composite ( Fig. 6 ). Accordingly, two experimental aspects about BNT–6BT:0.3ZnO should be emphasized. One is that the butterfly-shaped bipolar S – E curves and the non-zero negative strain confirm the ferroelectric nature, that is, there is no depolarization of this composite up to 125 °C, consistent with the ferroelectric results provided in Fig. 4 . The other is the temperature-independent unipolar strain value and the S max / E max : for the BNT–6BT:0.3ZnO, the unipolar strain increases from 0.11% at RT to 0.12% at 125 °C, and the corresponding S max / E max increases from 157 pm V −1 at RT to 171 pm V −1 at 125 °C. However, for the BNT–6BT, the unipolar strain changes significantly from 0.11% at RT, 0.43% at 75 °C, to 0.26% at 125 °C, and the S max / E max changes from 180 pm V −1 at RT, 715 pm V −1 at 75 °C, to 500 pm V −1 at 125 °C. Clearly, the thermal stability of piezoelectric property of the BNT–6BT:0.3ZnO composite has been improved. This will provide opportunities for industrial application in the form of sensors and transformers, where device manufacture often entails temperature treatment around 100 °C, which would lead to depolarization of the BNT–6BT piezoceramics. Again, the BNT–6BT:0.4ZnO composite has similar bipolar and unipolar S–E curves with BNT–6BT:0.3ZnO ( Supplementary Fig. 7 ). 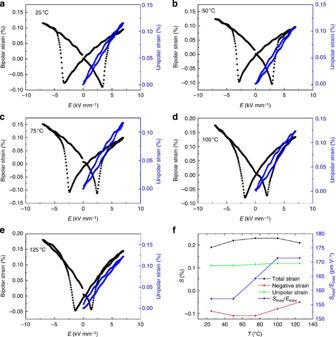Figure 6: Temperature-dependent bipolar and unipolarS–Ecurves of BNT–6BT:0.3ZnO composite. (a–e) The butterfly-shaped bipolarS–Ecurves again confirm the elimination of depolarization. (f) The corresponding temperature-dependent total strain, negative strain, unipolar strain andSmax/Emaxindicate that the temperature stability of the piezoelectric property has been improved vastly. Figure 6: Temperature-dependent bipolar and unipolar S–E curves of BNT–6BT:0.3ZnO composite. ( a – e ) The butterfly-shaped bipolar S–E curves again confirm the elimination of depolarization. ( f ) The corresponding temperature-dependent total strain, negative strain, unipolar strain and S max / E max indicate that the temperature stability of the piezoelectric property has been improved vastly. 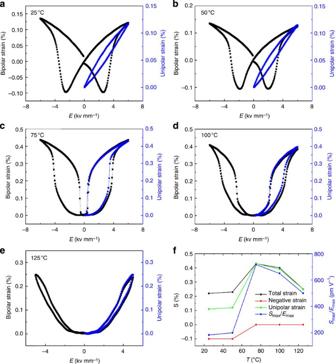Figure 7: Temperature-dependent bipolar and unipolarS–Ecurves of BNT–6BT solid solutions. (a–e) The disappearance of negative strain in bipolarS–Eand the suddenly increased total strain near 75 °C confirm the existence of depolarization. (f) The corresponding temperature-dependent total strain, negative strain, unipolar strain andSmax/Emaxindicate that the piezoelectric property of the solid solution is temperature sensitive, similar to its ferroelectric property. Full size image Figure 7: Temperature-dependent bipolar and unipolar S–E curves of BNT–6BT solid solutions. ( a – e ) The disappearance of negative strain in bipolar S–E and the suddenly increased total strain near 75 °C confirm the existence of depolarization. ( f ) The corresponding temperature-dependent total strain, negative strain, unipolar strain and S max / E max indicate that the piezoelectric property of the solid solution is temperature sensitive, similar to its ferroelectric property. Full size image To further confirm the elimination of thermal depolarization in the composites, the retained d 33 after thermal annealing of the BNT–6BT, BNT–6BT:0.3ZnO and BNT–6BT:0.4ZnO are depicted in Fig. 8 . The d 33 of the BNT–6BT decreases sharply from 110 pC N −1 at RT to 5 pC N −1 after exposure to 125 °C due to the well-known thermal depoling effect. However, this is not the case for the other two composites. For example, after exposure to 125 °C, BNT–6BT is almost thermally depoled, while the composites of BNT–6BT:0.3ZnO and BNT–6BT:0.4ZnO can well maintain their piezoelectric property. Here, the retained d 33 values are as high as 80 and 75 pC N −1 , respectively. 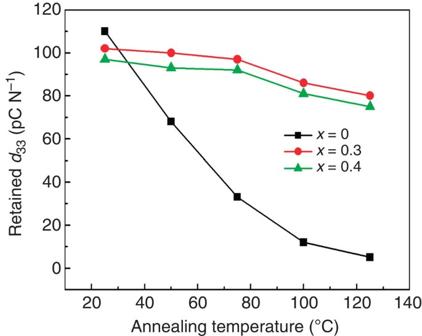Figure 8: The retainedd33of BNT–6BT, BNT–6BT:0.3ZnO and BNT–6BT:0.4ZnO as a function of annealing temperature. The BNT–6BT demonstrates depolarization-suppressedd33; at 125 °C the BNT–6BT is almost thermally depoled. However, both the BNT–6BT:0.3ZnO and BNT–6BT:0.4ZnO can retain their piezoelectric property withd33values of 80 and 75 pC N−1after annealing at 125 °C, respectively. Figure 8: The retained d 33 of BNT–6BT, BNT–6BT:0.3ZnO and BNT–6BT:0.4ZnO as a function of annealing temperature. The BNT – 6BT demonstrates depolarization-suppressed d 33 ; at 125 °C the BNT – 6BT is almost thermally depoled. However, both the BNT – 6BT:0.3ZnO and BNT – 6BT:0.4ZnO can retain their piezoelectric property with d 33 values of 80 and 75 pC N −1 after annealing at 125 °C, respectively. Full size image Although the origin of depolarization is still somewhat unclear, it is commonly believed that the size and charge disorder in BNT-based solid solutions decreases the ferroelectric order. BNT–6BT is classified as a nonergodic relaxor, which assumes long-range ferroelectric order after poling. Upon heating, it transits from an aligned domain structure to a randomized domain structure to an ergodic relaxor with polar nanoregions when it depolarizes [28] . Depolarization can be suppressed by an external poling field [34] , [35] : as the domains at the grain boundaries carry a misfit polarization, a depolarization field develops [36] ( Fig. 9a ). This depolarization field is at a maximum at pore surfaces and is considered to be 0.1 P r at grain boundaries in average [37] . After removing the poling field, this depolarization field leads to complete back-switching of the domains at T d ( Fig. 9b ). According to Jo et al. [28] , at zero electric field there exists a randomized domain structure. This mechanism is also consistent with the following fact: pure BNT–6BT and other BNT-based solid solutions always demonstrate the well-known pinched P–E loops with non-zero remnant polarization four-peak J–E curves, and zero negative-strain bipolar S–E curves above T d , as typical for relaxors (see Figs 5 and 7 ). 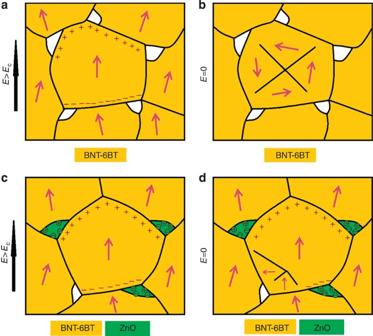Figure 9: The schematic of depolarization in BNT–6BT solid solution and that of suppressed depolarization in BNT–6BT:ZnO composite. (a,b) Domain schematics of BNT–6BT solid solution with and without an external poling field. With an applied poling field atTd, the polar nanoregions grow, leading to the appearance of large ferroelectric domains and a mismatch of polarization charges at the grain boundaries. However, after removing the poling field, the depolarization field destabilizes the ferroelectric domains. At the same time, the polarization charges decrease. All other poled grains have the similar depolarization behaviour. In addition, without ZnO, BNT–6BT solid solutions are not dense enough with some voids, as underpinned inSupplementary Fig. 3. (c,d) In the BNT–6BT:ZnO composite, the poling field will not only induce large ferroelectric domains and a mismatch of polarization charges at BNT–6BT/BNT–6BT grain boundaries, but also induce charges from semiconductor ZnO at the BNT–6BT/ZnO grain boundaries. The induced charges (circled) partially reduce the depolarization field. After removing the poling field, there is little back-switching as the depolarization field is only uncompensated at grain boundaries without ZnO. Therefore, the BNT–6BT:ZnO composite will not demonstrate depolarization behaviour. It is also noted that the distribution of ZnO at grain boundaries can reduce the porosity of the composite so that the relative density becomes higher compared with pure BNT–6BT. Figure 9: The schematic of depolarization in BNT–6BT solid solution and that of suppressed depolarization in BNT–6BT:ZnO composite. ( a , b ) Domain schematics of BNT – 6BT solid solution with and without an external poling field. With an applied poling field at T d , the polar nanoregions grow, leading to the appearance of large ferroelectric domains and a mismatch of polarization charges at the grain boundaries. However, after removing the poling field, the depolarization field destabilizes the ferroelectric domains. At the same time, the polarization charges decrease. All other poled grains have the similar depolarization behaviour. In addition, without ZnO, BNT – 6BT solid solutions are not dense enough with some voids, as underpinned in Supplementary Fig. 3 . ( c , d ) In the BNT – 6BT:ZnO composite, the poling field will not only induce large ferroelectric domains and a mismatch of polarization charges at BNT – 6BT/BNT – 6BT grain boundaries, but also induce charges from semiconductor ZnO at the BNT – 6BT/ZnO grain boundaries. The induced charges (circled) partially reduce the depolarization field. After removing the poling field, there is little back-switching as the depolarization field is only uncompensated at grain boundaries without ZnO. Therefore, the BNT – 6BT:ZnO composite will not demonstrate depolarization behaviour. It is also noted that the distribution of ZnO at grain boundaries can reduce the porosity of the composite so that the relative density becomes higher compared with pure BNT – 6BT. Full size image The mechanism in the BNT–6BT:0.3ZnO composite is a very novel one. We therefore can only provide the following hypothesis: An external poling field leads to the alignment of ferroelectric domains in BNT–6BT grains and unbound misfit compensation charges at BNT–6BT/BNT–6BT grain boundaries. It further provides mobile electronic charges from semiconductor ZnO to distribute at the BNT–6BT/ZnO grain boundaries, as schematically depicted in Fig. 9c , in which the depolarization field is partially compensated by the charges stemming from ZnO. Therefore, even after removing the poling field, the BNT–6BT grains can still keep the poled states and will provide reduced back-switching as noted in Figs 3 and 9d . Useful computations on related effects in the fields of aging and fatigue have recently been advanced [37] . If we contemplate a full compensation of local polarization mismatch at grain boundaries, a charge separation h in ZnO grains would be required as: . Here, is the elemental charge, is the misfit polarization at grain boundaries [37] and is a concentration of electronic carriers in ZnO. If we take (ref. 38 ), then we arrive at . As the ZnO grain size was ascribed to be ~0.5 μm, partial charge compensation and hence, reduction of the local depolarization field is feasible. At the same time, the equation offers opportunities for future microstructural tailoring of ferroelectric composites to adjust the local depolarization fields. Further evidence that the depolarizing field hinders domain switching is afforded by studies on a comparison of electrical and mechanical domain switching. It is demonstrated that electrical switching requires substantially higher energies as compared with mechanical switching where depolarization fields are not created [39] . Here it must be emphasized that the 0–3-type composite microstructure is an important ingredient because if ZnO particles form a network path throughout the BNT–6BT matrix, the composite will demonstrate semiconductor behaviour and the sample will provide too high a conductivity. The above domain evolution process is consistent with the XRD results measured on unpoled and poled samples ( Supplementary Fig. 2 ). The poled BNT–6BT: x ZnO composites help to retain the tetragonal structure, revealing that domains in composites are not relaxed completely after removing the poling field, which is not the case for pure BNT–6BT. As far as the role of ZnO is concerned, we believe that ZnO offers one clear advantage: its semiconductor nature ensures that it can act as a charge pool, so it provides charges to form a field to partially compensate the depolarization field. If a dielectric insulator is introduced to form a composite with BNT–6BT, the depolarization behaviour cannot be suppressed since insulators cannot provide enough charges to form a local field to compensate the local depolarization field. To verify this idea, BNT–6BT: x ZrO 2 ( x =0~0.4) composites were also prepared and investigated. All electrical measurements confirm that BNT–6BT: x ZrO 2 composites depict depolarization behaviour like BNT-based solid solutions. The typical temperature-dependent ε r and tan δ are plotted in Supplementary Fig. 8 . There are two anomalies of ε r that correspond to T d and T m , respectively, and the sharp decrease of tan δ around 150 °C corresponds to T d . These experimental results support our model. In summary, we have designed and prepared semiconductor/relaxor 0–3-type composites BNT–6BT: x ZnO. Detailed microstructure analysis substantiates that ZnO particles are isolated from each other and occupy the grain boundaries of the BNT–6BT matrix. The composites exhibit excellent piezoelectric properties: first, the T d increases with increasing x , and the depolarization disappears around x =0.3. This is experimentally confirmed by systematical temperature-dependent dielectric, ferroelectric, piezoelectric measurements and temperature-dependent XRD measurements. Second, the introduction of ZnO can enhance electric properties and improve thermal stability, both of which are advantages for practical applications, particularly for sensors and transformers. Third, by further comparing with BNT–6BT: x ZrO 2 composites, the mechanism for the observations in BNT–6BT: x ZnO composites are rationalized based on the charge-order model. We believe that these results can provide a simple and effective way to defer the thermal depolarization to higher temperature, improve electrical property and thermal stability of conventional BNT-based and other lead-free piezoceramics, which may pave the way for applications. Furthermore, this work provides a referential method to develop novel piezoceramics with designed microstructures and optimized physical properties. We therefore expect innovative work in composites in the field of in situ diffraction, modelling of electric-field distributions and synthesis to optimize second-phase distribution and microstructure in general. Depolarization in single crystals versus polycrystalline materials may also highlight the role of the depolarization field. Sample preparation BNT–6BT was prepared independently. Stoichiometric Bi 2 O 3 (99.8%), BaCO 3 (99.0%), Na 2 CO 3 (99.8%) and TiO 2 (99.0%, all from Alfa Aesar), were weighed and ball milled in ethanol for 24 h. The dried slurries were calcined at 900 °C for 3 h with an increasing and decreasing ramp rate of 5 °C min −1 , ground by hand for 0.5 h, ball milled again in ethanol for 24 h, followed by a drying process. The powders were sintered in covered alumina crucibles at 1,100 °C for 3 h and then ground by hand for 1.0 h. In this way, single-phase BNT–6BT powders were obtained. Afterwards, both the prepared BNT–6BT powders and the commercial ZnO nanoparticles with the size of 25 nm (PlasmaChem, Germany) were weighed according to the formula of BNT–6BT: x ZnO with x= 0.1, 0.2, 0.3 and 0.4. Each mixture was ball milled again in ethanol for 24 h, dried and subsequently pressed into green disks with a diameter of 10 mm under 40 MPa. Sintering was carried out in covered alumina crucibles at 1,000–1,050 °C for 1.0 h with a rapid increasing and decreasing temperature rate of 9 °C min −1 The relatively low sintering temperature, short sintering time and rapid increasing/decreasing ramp rate were adopted to prevent the diffusion between ZnO and BNT–6BT and to suppress the growth of ZnO nanoparticles. For the x =0 composition, that is, BNT–6BT disks were sintered at 1,050 °C for 1.0 h with the heating and cooling rate of 9 °C min −1 for comparative investigations. The BNT–6BT: x ZrO 2 composites were prepared in the same way, and ZrO 2 (99.9%, Alfa Aesar) was used as the raw material. Crystal structure analysis The crystal structure of the composites was characterized by powder XRD with Cu K α1 source. RT XRD measurements on unpoled and poled (6.0 kV mm −1 for x =0 and 7.0 kV mm −1 for others, 20 min, RT) were carried out using Rigaku Ultima III, while temperature-dependent XRD measurements were performed using PANalytical, PW 3040-X’Pert Pro. The microstructures and element distribution were analysed by SEM (FEI Quanta 200 and Zeiss Ultra 55). Two-dimensional micro-Raman measurements (Horiba Jobin Yvon HR800) were carried out to confirm the composite microstructure. Electrical property measurements For electrical measurements, the circular surfaces of the ground disks with the diameter of ~8.5 mm and the thickness of ~0.5 mm were covered by a thin layer of silver paste and fired at 550 °C for 30 min. Dielectric constant ( ε r ) and loss factor (tan δ ) were measured using an impedance analyzer (HP4294A) at several frequencies in a temperature range from 30 to 320 °C on unpoled and poled samples. The P–E loops, J–E curves and S–E curves were measured at 1 Hz using the TF analyzer 1000 (AixACCT) in silicone oil with controllable temperature from RT (~25 °C) to 125 °C. The RT piezoelectric coefficient ( d 33 ) was measured on poled ceramics by a Berlincourt- d 33 -meter (ZJ-6A). To measure the effect of thermal annealing on d 33 , the ceramics were poled at RT (6.0 kV mm −1 for x =0 and 7.0 kV mm −1 for other compositions, 20 min) and annealed at different temperatures (25–125 °C with step of 25 °C) for 10 min and then the retained d 33 was determined after the poled ceramics were cooled down to RT. These crucial experiments were repeated several times. How to cite this article: Zhang, J. et al. Semiconductor/relaxor 0–3-type composites without thermal depolarization in Bi 0.5 Na 0.5 TiO 3 -based lead-free piezoceramics. Nat. Commun. 6:6615 doi: 10.1038/ncomms7615 (2015).